Dislocation motion and grain boundary migration in two-dimensional tungsten disulphide Dislocations have a significant effect on mechanical, electronic, magnetic and optical properties of crystals. For a dislocation to migrate in bulk crystals, collective and simultaneous movement of several atoms is needed. In two-dimensional crystals, in contrast, dislocations occur on the surface and can exhibit unique migration dynamics. Dislocation migration has recently been studied in graphene, but no studies have been reported on dislocation dynamics for two-dimensional transition metal dichalcogenides with unique metal-ligand bonding and a three-atom thickness. This study presents dislocation motion, glide and climb, leading to grain boundary migration in a tungsten disulphide monolayer. Direct atomic-scale imaging coupled with atomistic simulations reveals a strikingly low-energy barrier for glide, leading to significant grain boundary reconstruction in tungsten disulphide. The observed dynamics are unique and different from those reported for graphene. Through strain field mapping, we also demonstrate how dislocations introduce considerable strain along the grain boundaries and at the dislocation cores. Dislocations can significantly modulate the electronic properties of crystals by introducing states within their band gap [1] . They can act as nucleation sites for the onset of deformation, when subjected to stress [2] , [3] , [4] . When exposed to chemical functional groups, defects can also behave as highly reactive sites and efficiently trap different molecules [5] , [6] . A rich variety of dislocations have recently been observed in 2D crystals such as graphene, hexagonal boron nitride and transition metal dichalcogenides (TMDs) [7] , [8] , [9] , [10] , [11] , [12] . Due to the high surface to volume ratio of 2D crystals, dislocations can lead to unique crystal geometries by introducing strain [9] . Dislocation migration in three-dimensional bulk crystals occurs when a large number of atoms move simultaneously along or perpendicular to its Burgers vector, leading to glide or climb, respectively. In contrast to bulk crystals, dislocation migration in 2D crystals can take place through the movement of few atoms near the dislocation core and the massive movement of atoms is not required. Because of the unusual geometry of 2D crystals, dislocation glide occurs by the movement of atoms on the surface, in which atomic diffusion typically has a lower-energy barrier when compared with the bulk. Graphene is an example of a 2D crystal, in which a dislocation glide can take place through Stone–Wales bond rotation [7] , [9] , [13] , [14] . Unlike graphene, MX 2 TMDs consist of metal (for example, M=Mo, W, Nb and so on) atoms sandwiched by chalcogen atoms (for example, X=S, Se, Te) establishing partial ionic bonds (see Supplementary Fig. 1 ). This elemental heterogeneity can give rise to a completely different migration behaviour as homo-nuclear bond formation is not energetically favourable. In this study, we use aberration-corrected scanning transmission electron microscopy (STEM) imaging to probe the dislocations and their migration mechanisms leading to grain boundary migration in WS 2 monolayer. We study the grain boundary structure, stability and dynamics resulting from the sample-beam interactions in chemical vapor deposition (CVD) grown monolayer WS 2 (ref. 15 ). With a combination of experiment and theory, this investigation elucidates for the first time the dislocation-motion mechanisms in a hetero-elemental WS 2 2D crystal and the local strain field associated with its dislocations. 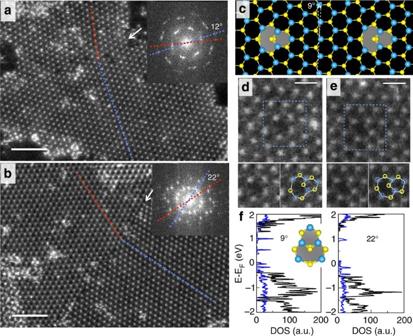Figure 1: Low- and high-angel grain boundary structure of the monolayer WS2with its electronic structure. (a) ADF-STEM image of a tilt grain boundary in a single-layer WS2sheet and the corresponding FFT, with a misorientation angle of 12° between two grains as marked by dashed lines. Scale bar, 2 nm. (b) ADF-STEM image and the corresponding FFT of a grain boundary with a 22° misorientation angle. Scale bar, 2 nm. (c) Atomic structure model calculated from first principles for a 9° grain boundary composed of 6|8 dislocations. (d,e) The magnified regions of a 6|8 dislocation core in 12° and 22° grain boundaries, respectively. The lower images highlight the position of W and S atoms and the 6|8 dislocation structure. The scale bar is 5 Å. (f) Total electronic density of states (grey line) for the 9° (left) and 22° (right) grain boundaries composed of 6|8 structures, respectively. The blue line shows the states contributed by atoms forming the dislocations. Grain boundary structure in a monolayer WS 2 and its electronic structure Figure 1a,b illustrates two tilt grain boundaries (shown by the arrows) with 12° and 22° misorientation angles in a monolayer of WS 2 exhibiting several 6|8 edge dislocations. At the larger tilt of 22°, a higher dislocation density is observed along the grain boundary that leads to higher local strain. Such level of strain near the grain boundaries can lead to a slight warping of the grains out of the WS 2 monolayer plane, resulting in the contrast loss of sulphur atoms in the annular dark field (ADF) STEM images as a result of local distortion (see Supplementary Figs 2 and 3 ). Both grain boundaries are dominantly comprised of 6|8 edge dislocations ( Fig. 1d,e ), which are derived from 5|7 defects by the insertion of a two-atom column of S between the W–W bonds [16] . In particular, the 6|8 dislocations are predicted to be more favourable under S-rich conditions when compared with 5|7 dislocations in TMDs [16] . 6|8 dislocations were also observed in MoS 2 (ref. 17 ) but have not been observed in any other 2D materials. The distance between dislocation cores along the 12° grain boundary is about 1 nm (see Supplementary Fig. 4 ), which is in close agreement with the simulated structure of the 9° grain boundary composed of 6|8s ( Fig. 1c ). Electronic structure analysis from first-principles calculations indicates that 6|8 dislocations introduce a series of localized states within the band gap of WS 2 monolayer ( Fig. 1f ), which may serve as sinks for charge carriers to undermine the electron transport in WS 2 . More importantly, the 6|8 dislocations are nonmagnetic, in contrast to the magnetic 5|7 dislocations in TMDs [18] . This indicates that the incorporation of two sulphur atoms in the 5|7 dislocations can quench the radical electronic states of the 5|7 dislocations and therefore electronically stabilize the 6|8 dislocations. This distinctly differentiates TMDs from graphene [19] , [20] , [21] and hexagonal boron nitride [10] , in which 5|7 dislocations are also observed. Figure 1: Low- and high-angel grain boundary structure of the monolayer WS 2 with its electronic structure. ( a ) ADF-STEM image of a tilt grain boundary in a single-layer WS 2 sheet and the corresponding FFT, with a misorientation angle of 12° between two grains as marked by dashed lines. Scale bar, 2 nm. ( b ) ADF-STEM image and the corresponding FFT of a grain boundary with a 22° misorientation angle. Scale bar, 2 nm. ( c ) Atomic structure model calculated from first principles for a 9° grain boundary composed of 6|8 dislocations. ( d , e ) The magnified regions of a 6|8 dislocation core in 12° and 22° grain boundaries, respectively. The lower images highlight the position of W and S atoms and the 6|8 dislocation structure. The scale bar is 5 Å. ( f ) Total electronic density of states (grey line) for the 9° (left) and 22° (right) grain boundaries composed of 6|8 structures, respectively. The blue line shows the states contributed by atoms forming the dislocations. Full size image Strain-field mapping of the grain boundaries in the monolayer WS 2 Dislocations at grain boundaries can locally introduce considerable levels of strain that can further accommodate dislocation movements in 2D crystals. Here we use geometric phase analysis [22] to map the strain fields at the dislocation cores in the low- and high-angle grain boundaries. A symmetric strain matrix was used to obtain strain fields for ε xx , ε xy , ε yy and rotation xy ( Fig. 2 ). 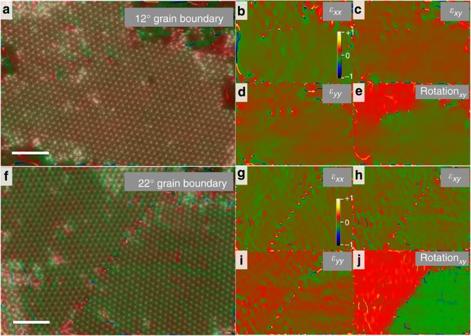Figure 2: Strain-field mapping of the low- and high-angle grain boundaries of the monolayer WS2. (a) A superimposed image of the 12° grain boundary and itsεxystrain map. Scale bar, 2 nm. (b)εxx, (c)εxy, (d)εyyand (e) rotationxymaps for the 12° grain boundary. (f) A superimposed image of the 22° grain boundary and its corresponding strain fieldεxy. Scale bar, 2 nm. (g)εxx, (h)εxy, (i)εyyand (j) rotationxymaps for the 22° grain boundary. The strain colour scale (shown inFig. 2b,g) corresponds to a range from −1 (black) to +1 (white), in which the boundary between red and green signifies 0. Figure 2a,f shows superimposed images of the 12° and 22° grain boundaries (originally depicted in Fig. 1a,b , respectively) and their ε xy strain maps, indicating a considerable amount of shear strain present at the dislocation cores. Figure 2b–e and g–j , shows ε xx , ε xy , ε yy strain and rotation xy maps for the 12° and 22° grain boundaries, respectively. The 12° grain boundary shows shear strain ( ε xy ) in the range of 5–25% (corresponding to distances ranging from 0.50 to 0.035 nm from the dislocation core), whereas a considerably higher strain ranging from 5 to 58% (corresponding to distances ranging from 0.50 to 0.035 nm from the dislocation core) was found for the 22° grain boundary. In addition, the 22° grain boundary shows larger ε xx , ε yy strain fields and lattice rotation xy compared with the 12° grain boundary (see also real space strain analysis in Supplementary Fig. 5 ). Such high-strain fields associated with the dislocations can lead to unique migration dynamics and reconstruction mechanisms that need to be further explored. Figure 2: Strain-field mapping of the low- and high-angle grain boundaries of the monolayer WS 2 . ( a ) A superimposed image of the 12° grain boundary and its ε xy strain map. Scale bar, 2 nm. ( b ) ε xx , ( c ) ε xy , ( d ) ε yy and ( e ) rotation xy maps for the 12° grain boundary. ( f ) A superimposed image of the 22° grain boundary and its corresponding strain field ε xy . Scale bar, 2 nm. ( g ) ε xx , ( h ) ε xy , ( i ) ε yy and ( j ) rotation xy maps for the 22° grain boundary. The strain colour scale (shown in Fig. 2b,g ) corresponds to a range from −1 (black) to +1 (white), in which the boundary between red and green signifies 0. Full size image In this report, we show a qualitatively new phenomenon on the structural dynamics of dislocations in 2D TMDs: the migration of 6|8 dislocations in a monolayer WS 2 at room temperature and low-accelerating voltage (80 kV) for both low- and high-angle grain boundaries. Dislocation migration in a 12° grain boundary of the monolayer WS 2 Supplementary Movie 1 shows a series of ADF-STEM images where dislocation migration leads to grain boundary motion in a monolayer of WS 2 . Selected snapshots from the observed atomic-scale dynamics can be seen in Fig. 3 . The consecutive frames of this movie are 5 s apart, showing the dislocation migration in a low-angle grain boundary (12°). 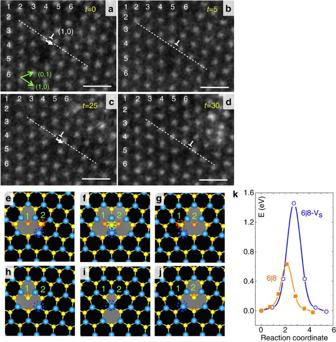Figure 3: Dislocation migration in a 12° grain boundary. Dislocation glide along its Burgers vector (1,0) on its glide plane (shown by dashed lines) fromatob. Several seconds later the same dislocation glides again along (1,0) fromctod. (e–g) Structural models for the migration of a 6|8 dislocation with one S vacancy (6|8-VS). (h–j) 6|8 with initial, saddle-point and final structures in the left, middle and right panels, respectively. (k) Minimum energy paths during migration for two dislocation cores. The scale bars are 6 Å. Figure 3a,b shows glide of the marked dislocation to the bottom right, along its Burgers vector. Figure 3c,d reveals the same dislocation several seconds later, which moves to the bottom right again, through a glide along its Burgers vector marked by an arrow in Fig. 3c . These dynamics are analysed by considering the dislocation core with respect to a stationary vacancy as a reference point in every frame (see Supplementary Fig. 6 ). By comparing individual frames of the movie, S atoms are observed to be very dynamic and mobile around the dislocation cores. This dynamic behaviour could lead to dislocations exhibiting S-rich or -deficient conditions as well as different atomic arrangements [23] . In particular, S-rich/deficient structures were observed at the dislocation core, which can be achieved by either thermodynamically controlling the chemical potential [16] or by knock-on displacement of atoms from the incident electron beam [17] , [24] , [25] . A S-rich structure with two sulphur atoms at the dislocation core can form a 6|8 dislocation (see Fig. 3a and Supplementary Figs 7A and 8C ), whereas a S-deficient structure ( Fig. 3c and Supplementary Figs 7B and 8F ) with one S atom missing at the dislocation core can result in the formation of a 6|8-V S dislocation (6|8 dislocation with one sulphur vacancy). Here the formation of S vacancies in TMDs results from the electron beam-sample interactions at 80 kV (ref. 24 ). When using this particular electron beam energy, we are on the edge of the knock-on threshold, where W atoms mainly remain in the lattice, whereas several S vacancies can be created at the edges, dislocations and within the defect-free region of the monolayer. Sulphur adatoms arising from this knock-on process can display mobility on the surface of the WS 2 monolayer, especially around the dislocation cores and edges. In addition, other adatoms, such as carbon, can exhibit similar mobility and interaction with the dislocations, which should be further investigated. Such dynamics are the key component for transforming the dislocation structure leading to dislocation glide and grain boundary migration [9] , [26] . Figure 3: Dislocation migration in a 12° grain boundary. Dislocation glide along its Burgers vector (1,0) on its glide plane (shown by dashed lines) from a to b . Several seconds later the same dislocation glides again along (1,0) from c to d . ( e – g ) Structural models for the migration of a 6|8 dislocation with one S vacancy (6|8-V S ). ( h – j ) 6|8 with initial, saddle-point and final structures in the left, middle and right panels, respectively. ( k ) Minimum energy paths during migration for two dislocation cores. The scale bars are 6 Å. Full size image First-principles calculations were carried out in order to gain a better understanding of the dislocation migration mechanism observed in WS 2 monolayer. Both dislocation structures, 6|8 and 6|8-V S , can be formed through interaction of the 5|7 dislocations with S interstitials [16] , [27] . Figure 3e–j depicts the mechanism for the migration of the 6|8-V S and 6|8 dislocations. In this figure, the orange atoms located at the dislocation core show the S atoms on the bottom layer, whereas the yellow atoms indicate S atoms on the top layer. The migration of 6|8-V S is displayed in Fig. 3e–g with only one S atom at site 1. Our calculations suggest dislocation migration starts when one of the top S atoms at site 2 (red dashed circle) moves to site 1. This movement is accompanied by the circled W atom simultaneously gliding and disconnecting from the S atom at site 2, thus creating a bond with the S atom at site 1. The concurrent movements of W and S atoms lead to a significant structural distortion in the saddle-point structure ( Fig. 3f ) that results in a migration barrier of about 1.4 eV. This energy barrier is considerably lower than the diffusion energy barrier for a single S vacancy (V S ), which is estimated to be 2.3 eV for MoS 2 of the same lattice [28] , highlighting the important role of the dislocations and their interaction with S vacancies in mediating both the dislocation and S migration in TMDs through the coupled displacement of W atoms. Without the S vacancy in the dislocation core ( Fig. 3h–j ), the dislocation migration barrier further drops to 0.6 eV ( Fig. 3k ). Under this condition, the lattice undergoes a much smaller structural distortion, as the S sublattice recovers and only a single W atom is involved during the dislocation glide through direct bond breaking and reconnection. As shown in Fig. 3h–j , the circled W atom breaks its bonds with S atoms at site 2, and reconnects with S atoms at site 1. As the glide proceeds, a W-oriented 4|6 structure forms at the saddle point with the (circled) W-S bond length increased by about 20 pm compared with those forming hexagons ( Fig. 3i ). This results in a considerable drop in the energy barrier for dislocation glide under S-rich conditions. Such a low-migration barrier in monolayer WS 2 is already similar to bubbles diffusing in liquids, and in sharp contrast to graphene, where there is an energy barrier of 5–10 eV for dislocation glide through bond rotation [9] , [13] , [14] . Other TMD systems can exhibit similar migration mechanisms to WS 2 because of their similar bonding and atomic structure. Dislocation migration in a 22° grain boundary of the monolayer WS 2 Supplementary Movie 2 shows dislocation migration in a high-angle (22°) grain boundary in monolayer WS 2 . A sequence of ADF-STEM images from the dislocation cores can be followed in Fig. 4a–d (see Supplementary Fig. 9 for Burgers circuit analysis and Supplementary Fig. 10 for the relaxed dislocation structures). The grain boundary in this area is composed of both 6|8 dislocations with (1, 0) Burgers vector and 4|6 dislocations with (1, −1) (equivalent to (0, 1)) [16] Burgers vector (see Fig. 4e ). In the high-angle grain boundaries with a higher density of dislocations, the migration of different dislocations can be coupled together, resulting in different migration paths. 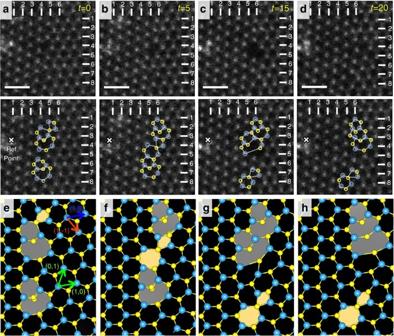Figure 4: Dislocation migration in a high-angle 22° grain boundary. A sequence of ADF-STEM images showing the migration of the dislocation cores in a 22° GB (a–d) with their corresponding structural models (e–h). One 4|6 and two 6|8 dislocations (a) further migrate through glide and climb (b). 10 s later, two side-by-side 6|8s (c) recombine to form a 6|6|8 dislocation (d). The green arrows ineshow the crystal vectors for the pristine lattice, whereas the blue and orange arrows indicate two Burgers vectors (1, 0) and (1, −1) (equivalent to (0, 1)) for 6|8 and 4|6, respectively. The scale bars are 7 Å. Figure 4a,b reveals two consecutive frames of the grain boundary 5 s apart. The top and bottom 6|8 dislocations glide two and one steps along the (1, 0) direction, respectively. Meanwhile, the 4|6 dislocation glides one step along the (1, −1) direction and then climbs one step in the (0, −1) direction. This migration results from the successive diffusion of few atoms locally near the 6|8 and 4|6 composite dislocations (see Supplementary Fig. 11 ). Here, for the first time, we show climb and glide as two representative migration paths for dislocation migration in 2D TMDs materials. Figure 4: Dislocation migration in a high-angle 22° grain boundary. A sequence of ADF-STEM images showing the migration of the dislocation cores in a 22° GB ( a – d ) with their corresponding structural models ( e – h ). One 4|6 and two 6|8 dislocations ( a ) further migrate through glide and climb ( b ). 10 s later, two side-by-side 6|8s ( c ) recombine to form a 6|6|8 dislocation ( d ). The green arrows in e show the crystal vectors for the pristine lattice, whereas the blue and orange arrows indicate two Burgers vectors (1, 0) and (1, −1) (equivalent to (0, 1)) for 6|8 and 4|6, respectively. The scale bars are 7 Å. Full size image Figure 4c shows the same dislocation after 10 s, in which two side-by-side 6|8 dislocations are formed as a result of further rearrangement of atoms around the composite dislocations during the dislocation climb. The two side-by-side 6|8 dislocations further merge through glide and form a 6|8|8 dislocation with (2, 0) Burgers vector, as shown in Fig. 4d . This dislocation glide is energetically favourable and leads to a significant energy release (about −2.4 eV). Such a large dislocation can create a high-strain field and is considered as an ideal site for S interstitials or other adatoms, such as C. The simultaneous climb and glide observed here is complex and different from the migration behaviour at low-angle grain boundaries, where dislocation migration is identified as an isolated glide process. Using aberration-corrected electron microscopy coupled with first principles calculations this study reveals unique and fascinating dislocation structures along the grain boundaries and their local strain fields in a monolayer of WS 2 . Strain analysis shows large levels of strain along the grain boundaries and locally at the dislocation cores. Through a series of ADF-STEM images, the movement of individual atoms have been successfully probed at the grain boundaries and within the dislocation cores. Owing to the unique geometry of 2D crystals, dislocations reside at the crystal surface and can easily interact with the surface atoms. Highly mobile S atoms can interact with the dislocation cores and form different derivative dislocation structures with different migration mechanisms involving the rearrangement of the local W and S atoms around the defect. We observe such dynamics to have a strikingly low-energy barrier leading to significant grain boundary reconstruction in TMDs, despite their complex lattice structure. Controlling defects such as grain boundaries and dislocations using electron or ion irradiation have important implications in the design of 2D materials with desired physicochemical properties, and this account has provided important pieces of information regarding the transformation of defects and their dynamics. Synthesis WS 2 synthesis was carried out through a two-step process [15] . Si wafers with a thermally deposited SiO 2 layer 285-nm thick were thoroughly cleaned with a piranha solution at 80 °C for at least 40 min. After piranha treatment, the Si/SiO 2 wafers were loaded in the chamber of a physical vapour deposition apparatus, PVD75 (Kurt J. Lesker). A 1-nm layer of WO 3 was thermally evaporated and deposited on the wafers at low pressures (10 −5 –10 −6 Torr). The Si/SiO 2 /WO 3 wafers were subsequently loaded into a quartz reaction tube for thermal treatment under a S environment. The pressure in the chamber was set to 35 mTorr for 10 min and of ultra high purity (UHP) Ar (30 s.c.c.m.) was then allowed to flow into the reaction tube, reaching a pressure of 250 mTorr. The split furnace was then heated to 850 °C. Transmission electron microscopy sample preparation The WS 2 films were transferred onto Quantifoil Au TEM grids by using a poly(methyl methacrylate) (PMMA)-assisted technique. The films were coated with a thin layer of poly(methyl methacrylate), which was cured at room temperature for at least 2 h. The samples were then immersed in hydrofluoric acid for a few seconds in order to lift off the PMMA-WS 2 films. The film was removed and immersed in five beakers of deionized water, subsequently. The film was then picked up by the TEM grid from the surface of the water and was dried for a few hours. The PMMA layer was dissolved in acetone and isopropanol. To remove the remaining contaminants, the grids were annealed under Ar atmosphere at 400 °C for 4 h. The residue of the PMMA formed a defected graphene film that served as a support during imaging of the flake. Imaging of grain boundary structure and dynamics TEAM I at the National Center for Electron Microscopy at Lawrence Berkeley National Laboratory was used for this study. ADF-STEM images of WS 2 were recorded using 80 kV, 70 pA of beam current, 30 mrad convergence semi-angle and an ADF semi-angle of ~45 mrad. Image pixel sizes were 25 pm and dwell time was 15 μs to provide sufficient time resolution to study grain boundary and defect migration dynamics. Density functional theory calculations Density functional theory (DFT) calculations have been performed with the Perdew–Burke–Ernzerhof parametrization [29] of the generalized gradient approximation and projector-augmented wave potentials [30] , [31] , using the Vienna Ab-initio Simulation Package [32] , [33] . The vacuum layer thickness is chosen to be larger than 10 Å to keep the spurious interaction negligible by adopting a supercell approach. Based on the plane-wave-based total energy minimization [34] , all structures are fully relaxed until the force on each atom was less than 0.01 eV Å −1 . The climbing image nudged elastic band method [35] was used to calculate the activation barrier with a convergence criterion of 0.1 eV Å −1 , which shows a negligible barrier difference when compared with those with a more stringent criterion of 0.05 eV Å −1 . All the structures have been constructed in nanoribbon configurations, and the strain effects have been examined (see Supplementary Figs 12 and 13 ). Although the tensile strain is shown to have little influence on the migration barrier ( Supplementary Fig. 12 ), shear strain results in the distortion of 6|8 cores, as observed in TEM images ( Supplementary Fig. 13 ). How to cite this article : Azizi, A. et al. Dislocation motion and grain boundary migration in two-dimensional tungsten disulphide. Nat. Commun. 5:4867 doi: 10.1038/ncomms5867 (2014).